Athermal photofluidization of glasses Azobenzene and its derivatives are among the most important organic photonic materials, with their photo-induced trans–cis isomerization leading to applications ranging from holographic data storage and photoalignment to photoactuation and nanorobotics. A key element and enduring mystery in the photophysics of azobenzenes, central to all such applications, is athermal photofluidization: illumination that produces only a sub-Kelvin increase in average temperature can reduce, by many orders of magnitude, the viscosity of an organic glassy host at temperatures more than 100 K below its thermal glass transition. Here we analyse the relaxation dynamics of a dense monolayer glass of azobenzene-based molecules to obtain a measurement of the transient local effective temperature at which a photo-isomerizing molecule attacks its orientationally confining barriers. This high temperature ( T loc ~800 K) leads directly to photofluidization, as each absorbed photon generates an event in which a local glass transition temperature is exceeded, enabling collective confining barriers to be attacked with near 100% quantum efficiency. The possibility of athermal photofluidization of a highly viscous medium can be understood using Maxwell’s intuitive picture for viscosity [1] , or its contemporary embodiments [2] , [3] expressed by η = G/ν , giving viscosity as the ratio of a typical modulus for local shear deformation G and ν , the average rate per molecule in equilibrium for randomly occurring local structural deconfinement/relaxation events. With a shear displacement applied, these events relax the associated stress once each local region has participated, taking ~10 −12 s in a low-viscosity fluid. In glasses, the viscosity is very high: events are limited by energy barriers large enough to make the event rate correspondingly very low ( ν <1/s in some cases), affording the possibility of reducing the viscosity if ν can be externally augmented. This may be achieved by photon absorption events, for example, which also occur at random, at a rate proportional to the intensity of incident light. Photon absorption deposits energy into a molecule, a localized thermal/mechanical impulse that spreads with time and dissipates in energy density. The effectiveness with which photons can generate local structural rearrangement (fluidization) events contributing to the increase of ν depends on the details of such a process, and can be expressed as a quantum efficiency for local fluidization, 0< QELF <1. If each absorbed photon contributes ( QELF ~1) then macroscopic photofluidization is readily achievable, with many orders of magnitude of viscosity reduction possible at light intensities that produce negligible thermal heating. Apparently, given its rarity, photofluidization occurs only under certain limited conditions, but its observation in azobenzene-based systems, such as doped polymers, at temperatures ~100 K below their glass transition [4] , [5] , [6] , [7] , indicates that high QELF may be a general feature of azobenzenes. Furthermore, this suggests that it may be high QELF in itself that enables the sensitive photo-phenomena observed in azobenzene-based solutions [8] , [9] , polymers [10] , monolayers [11] and inorganic glasses [12] , [13] , and their application to photo-control of molecular orientation, macroscopic material transport and mechanical deformation [4] , [5] , [14] , [15] . These questions are explored here in an experimental study of photo-manipulation of orientational order in an aminoazobenzene-based tethered self-assembled monolayer (SAM) glass, showing efficient induction of orientational order by exposure to linearly polarized light and dramatic lowering of orientational viscosity by unpolarized light. A picture of the photo-orientation process emerges in which isolated photoisomerization events attack distinct local and collective barriers at transient temperatures that are high enough ( T loc ~800 K) for each absorbed photon to induce a local glass transition, a fluidization event on the 1-nm 10-ps spacetime scale, that melts the local barriers, enabling attack of the collective barriers with unit quantum efficiency ( QELF ~1). Effectively complete bypass of the thermal process occurs at light intensity sufficiently low to produce no observable effects of average heating. The success of azobenzenes in converting photon energy to effective local fluidization can be attributed to their distinctive photo-induced change in molecular shape [16] , [17] , combined with, importantly, relatively slow (~10 ps) dynamics [18] of the resulting energy transfer to their local environment. Photomanipulation of an aminoazobenzene SAM The azo system studied (dMR) is the derivative of the dye methyl red [19] shown in Fig. 1a , synthesized and covalently bonded onto glass substrates to form dense, photoactive, SAMs, as sketched in Fig. 1b . Illumination of azobenzenes by polarized light produces anisotropic molecular orientation, as the molecules tend to align along the direction for which photo-randomization of their orientation is minimized, that is, with trans–cis photoexcitation transition moments (approximately the molecular long axis) normal to the incident polarization [20] , [10] , [11] . We have studied the photoalignment and relaxation of dMR SAMs by transiently exposing them to polarized 514-nm light and measuring the dynamics of the resulting in-plane birefringence at 632 nm using a high sensitivity polarimeter [21] . Two 514-nm actinic beams, one linearly polarized pump (LP, in-plane polarization p ) and one circularly polarized (CP) pump, illuminate the sample at near-normal incidence and can be switched on and off with 40-μs response time using ferroelectric liquid crystal electro-optical shutters. 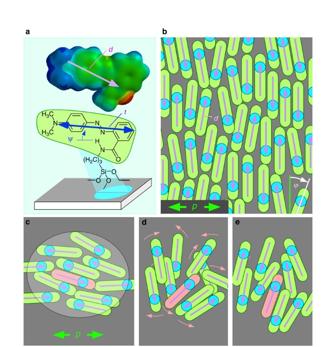Figure 1: The dMR self-assembled tethered molecular monolayer. (a) dMR molecular structure as synthesized and bonded to the glass, showing the VDW surface of the azo chromophore core, the molecular dipole momentd(pink), and the azo core long axis and chromophore transition momentt(blue). The angle between the core axis and surface plane isψ≈25°. (b) Sketch of in-plane structure with an in-plane orientation resulting from incident light polarized alongp(green arrow), showing the VDW projections of the dMR cores onto the surface plane (yellow green), the attachments of the tethers to the surface (cyan), the dipole orientationdand its azimuthal orientationφ. This sketch represents well the experimental average areal density. (c–e) All photo-induced changes in the dMR SAM are due to isolated events in which the absorption of a single photon of the polarization indicated excites a molecule (pink) causing isomerization and reorientation. (d) Because of the tethers, neighbouring molecules must pass over one another or squeeze past nearby tethers, leading to a local oriented, glassy state stabilized by a large barrierUth~kB(7,500 K). Isolated photon absorption produces such events with quantum efficiencyQELF~1 (one event/photon absorbed/molecule) because photo-induced barrier attack is atT=800 K, exceeding the glass transition for such local reorientation. Figure 1: The dMR self-assembled tethered molecular monolayer. ( a ) dMR molecular structure as synthesized and bonded to the glass, showing the VDW surface of the azo chromophore core, the molecular dipole moment d (pink), and the azo core long axis and chromophore transition moment t (blue). The angle between the core axis and surface plane is ψ ≈25°. ( b ) Sketch of in-plane structure with an in-plane orientation resulting from incident light polarized along p (green arrow), showing the VDW projections of the dMR cores onto the surface plane (yellow green), the attachments of the tethers to the surface (cyan), the dipole orientation d and its azimuthal orientation φ . This sketch represents well the experimental average areal density. ( c–e ) All photo-induced changes in the dMR SAM are due to isolated events in which the absorption of a single photon of the polarization indicated excites a molecule (pink) causing isomerization and reorientation. ( d ) Because of the tethers, neighbouring molecules must pass over one another or squeeze past nearby tethers, leading to a local oriented, glassy state stabilized by a large barrier U th ~ k B (7,500 K). Isolated photon absorption produces such events with quantum efficiency QELF ~1 (one event/photon absorbed/molecule) because photo-induced barrier attack is at T =800 K, exceeding the glass transition for such local reorientation. Full size image The methyl red core of dMR is attached to the glass surface by a short alkyl unit of four single C–C bonds, which gives an average angle between the long axis of the core and the surface plane of ψ ~25°, shown in Fig. 1a [22] , [19] , and permits reorientation and ~1-nm translation of the core. Figure 1b sketches the geometry of a locally oriented state with the molecules represented by rods having azimuthal orientation φ and a length-to-width ratio corresponding to the footprint of the van der Waals (VDW) shape of the core in Fig. 1a , with the tethers randomly attached to the surface, at locations represented by the blue circles. Optical absorbance measurements ( Supplementary Note 1 ) give a surface area/molecule of S =0.55 nm 2 . Comparison with the VDW footprint area of S m =0.45 nm 2 in Fig. 1b shows that the monolayer is densely packed, with the n-π* π-π* transition moments, represented by t , substantially parallel to the interface plane ( Fig. 1a ). In-plane orientation was induced in the monolayers by LP illumination such that the probe polarization and the in-plane average long molecular axis, the director n ≡ t ( φ ) , were at +45° and −45° from LP polarization, respectively. In this geometry the induced in-plane birefringence Δ n can be obtained from the transmission T through the crossed probe analyser using Δ n ( λ / πd ) T 1/2 , where d =0.5 nm is the mean thickness of the azo core, taken to be the SAM film thickness, ( Supplementary Methods , Supplementary Figs S1 and S2 ). The ultra-low polarimeter leakage at extinction, T min =2.4 × 10 −10 , enables measurement of in-plane SAM birefringence as small as Δ n ~0.001. During the illumination of a dMR SAM, initially randomized in orientation by thermal fluctuations, with the LP pump beam, starting at t =0, the in-plane birefringence Δ n ( t ) Δ n ( t )= n || — n ┴ , where n || (┴) is the index for polarization parallel (normal) to n , increases with increasing incident optical fluence, F (energy/area) from some small initial background value Δ n <~ 0.001, to Δ n ~0.14, as shown in Fig. 2a and Supplementary Fig. S4 . This birefringence can be attributed to in-plane ordering of the trans isomers, as they have larger optical polarizability anisotropy than the cis [23] , and generally larger anisotropy in their orientational distribution under conditions of orientational hole burning ( Supplementary Notes 2 and 3 ) [24] , [25] , [26] . The birefringence Δ n , which is proportional to the two-dimensional (2D) orientational order parameter S =<cos 2 φ —sin 2 φ >, indicates the development of in-plane ordering with S ~0.5, based on comparison of our measured Δ n with that of bulk azo-based nematics [27] . The Fig. 2a inset shows that SAM birefringence depends only on absorbed fluence (absorbed energy/area), F A , and that the initial growth of Δ n ( t ) is rather rapid, with the order of SAM being substantially developed at an absorbed fluence of F A ~1 photon absorbed per molecule (1 pa/mol), as calculated from the measured optical absorbance of 514 nm light incident on an isotropic SAM. Note that F A =1 pa/mol at F =20 mJ cm −2 ( Supplementary Note 1 ) [19] . 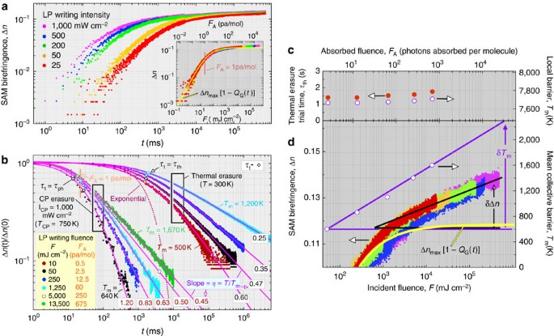Figure 2: Dynamics of writing and erasure of SAM in-plane birefringence Δn(t). (a)Δn(t) induced by LP light switched on att=0. Inset:Δn(t) depends only on average absorbed energy/areaFA, and atFA=1 photon absorbed per molecule (1 pa/mol), a substantial fraction of the saturated order is achieved. The solid yellow line isΔn(t) fromQG(t) (Equation 2). The nearly linear growth ofΔn(F) at lowFis the incremental accumulation inΔnfrom a stream of single-photon local alignment events, isolated and random in spacetime. (b) Measured decay ofΔn(t)/Δn(t=0) (solid symbols), initially written by LP light of varyingFand erased starting att=0 either thermally or by CP light of intensityICP=1 W cm−2.Δn(t)≈(t/τt)−ηat larget, and are fit well byQG(t) (solid curves), yielding the scaling timeτt, (diamonds, log–log plot ‘corner’), andη, the decay exponent. An exponential decay (purple dotted curve) is shown for comparison. The power law indicates an exponential distribution of collective barrier heights, withη=T/Tmthat decreases and thusTmthat increases with writingF. For eachF,ηis larger in the CP case, giving a larger effective temperature for CP erasure,TCP~750 K. For thermal erasure, the trial times for collective barrier crossing areτt~2 s (τtis labelled asτthin this regime), while for CP erasure at high CP intensityτph(ICP) occurs atFA=1 pa/mol (vertical orange lines) (τtis labelled asτph(ICP) in this regime). (c) Trial timesτt=τthand associated barriersTthfor local barrier crossing (collective barrier attempts) during thermal relaxation. Theτtdo not vary substantially with writingFAeven at lowFAwhere the writing events are isolated, indicating that they are determined by local constraints present in the unwritten SAM. (d) At largeFA,δΔn(FA) (black line) is the growth of Δn(FA) above the relaxation model prediction (yellow curve).δTm(FA) is the growth ofTmabove room temperature (purple line). The coupled logarithmic growth ofδΔnandδTmindicates ‘exhaustion’ or orientational ‘work hardening’ behavior52. Figure 2: Dynamics of writing and erasure of SAM in-plane birefringence Δ n ( t ). ( a ) Δ n ( t ) induced by LP light switched on at t =0. Inset: Δ n ( t ) depends only on average absorbed energy/area F A , and at F A =1 photon absorbed per molecule (1 pa/mol), a substantial fraction of the saturated order is achieved. The solid yellow line is Δ n ( t ) from Q G ( t ) (Equation 2). The nearly linear growth of Δ n ( F ) at low F is the incremental accumulation in Δ n from a stream of single-photon local alignment events, isolated and random in spacetime. ( b ) Measured decay of Δ n ( t) / Δ n ( t =0) (solid symbols), initially written by LP light of varying F and erased starting at t =0 either thermally or by CP light of intensity I CP =1 W cm −2 . Δ n ( t )≈( t/τ t ) − η at large t , and are fit well by Q G ( t ) (solid curves), yielding the scaling time τ t , (diamonds, log–log plot ‘corner’), and η , the decay exponent. An exponential decay (purple dotted curve) is shown for comparison. The power law indicates an exponential distribution of collective barrier heights, with η = T / T m that decreases and thus T m that increases with writing F . For each F , η is larger in the CP case, giving a larger effective temperature for CP erasure, T CP ~750 K. For thermal erasure, the trial times for collective barrier crossing are τ t ~2 s ( τ t is labelled as τ th in this regime), while for CP erasure at high CP intensity τ ph ( I CP ) occurs at F A =1 pa/mol (vertical orange lines) ( τ t is labelled as τ ph ( I CP ) in this regime). ( c ) Trial times τ t = τ th and associated barriers T th for local barrier crossing (collective barrier attempts) during thermal relaxation. The τ t do not vary substantially with writing F A even at low F A where the writing events are isolated, indicating that they are determined by local constraints present in the unwritten SAM. ( d ) At large F A , δ Δ n ( F A ) (black line) is the growth of Δ n ( F A ) above the relaxation model prediction (yellow curve). δT m ( F A ) is the growth of T m above room temperature (purple line). The coupled logarithmic growth of δ Δ n and δT m indicates ‘exhaustion’ or orientational ‘work hardening’ behavior [52] . Full size image Thermal and light-induced erasing: slow dynamics Figures 2b and 3a show Δ n ( t ) of anisotropic dMR-SAMs initially photowritten with LP light of the F and corresponding F A values displayed, and erased either by thermal fluctuations at T =300 K or by illumination with precisely CP light. Here t =0 is the time at which the LP beam is switched off, and the CP beam switched on in the photoerase case. These decay data reveal ultraslow, glassy relaxation, with no substantial decrease in the normalized orientational order Q ( t )=Δ n ( t )/Δ n (0) for t < τ t , the ‘corner’ on the log–log plot, obtained from the scaling time for the subsequent power law decay and indicated by the diamonds in Figs 2b and 3a . For the thermal case, τ t = τ th ~2 s and the power law decay at long time, Δ n ( t )/Δ n (0)~( t / τ th ) − η , is measurable out to several hours. The corner for thermal 2D XY orientational relaxation of comparably anisotropic but untethered molecules in freely suspended smectic C liquid crystal films is τ th ~10 −11 s ( Supplementary Note 4 ) [28] , [29] , [30] , [31] , [32] , [33] , suggesting, along with Fig. 1c–e , that two principal factors produce such slow orientational dynamics: (i) The high in-plane packing density, nearly that of the neat solid dye, promotes the tendency for the azo cores to associate by dipole and VDW interaction of their nearly planar chromophore cores, leading to strong in-plane structural correlations [34] that greatly enhance the energetic barriers preventing molecules from moving past one another. (ii) Local reorientation is limited by the tethers to discrete jumps as shown in Fig. 1c–e where in molecules must pass over or by one another, and to do so must either stretch or bend the tethers. 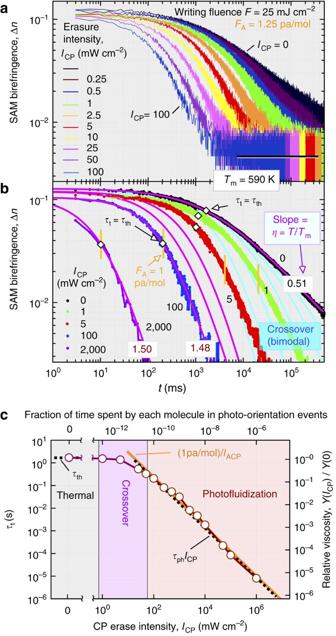Figure 3: Evolution from thermal to optical erasure of in-plane birefringence. (a) Variation of SAM birefringence relaxation with increasing erase intensity. The initial LP writing fluence is fixed atF=25 mJ cm−2. The rightmost data (black dots,ICP=0) show thermal erasure. The black solid line is the polarimeter leakage level, which has been subtracted out in (b). (b) Fits of selected relaxation data to the model (Equation 2; magenta curves). For the thermal decay (barrier attack temperatureT=300 K) the measuredη=0.51 shows the induced mean barrier height to beTm=590 K. At sufficiently highICPphoto-induced attempts are dominant and generate localT~800 K, independent ofICP. The fitted scaling (barrier attack) timesτt=τth, andτt=τph(ICP) are shown as diamonds. The decays are bimodal in the ‘crossover’ regime where the thermal and photo-induced trial times are comparable, with the solid cyan lines calculated from the relaxation model generalized for bimodal behaviour (Supplementary Equation S17). Vertical orange lines denoteFA=1 pa/mol. (c) Average inverse rateτtfor successful local molecular orientational barrier crossings and therefore for tests of the collective barriers to orientation, as a function of incident CP light intensityICP. At lowICP,τthas its thermal value (τt=τth~2 s), requiring ~1011room temperature molecular fluctuations to overcome aTth~7,500 K local barrier, while at highICPwe findτt~τph(ICP), which is nearly equal to (1 pa/mol)/IACP, whereIACPis the absorbed CP intensity (Supplementary Note 1,Supplementary Equation S2). This indicates that on average every absorbed photon generates a local barrier crossing test, evidence for a glass (fluidization) transition that obliterates the local barrier. This photo-induced bypass of the thermal trial process is responsible for the orientational photo-fluidization by CP illumination, directly manifested here as an orientational viscosity that decreases inversely with increasing intensity (γ1/ICP). Figure 3: Evolution from thermal to optical erasure of in-plane birefringence. ( a ) Variation of SAM birefringence relaxation with increasing erase intensity. The initial LP writing fluence is fixed at F =25 mJ cm −2 . The rightmost data (black dots, I CP =0) show thermal erasure. The black solid line is the polarimeter leakage level, which has been subtracted out in ( b ). ( b ) Fits of selected relaxation data to the model (Equation 2; magenta curves). For the thermal decay (barrier attack temperature T =300 K) the measured η =0.51 shows the induced mean barrier height to be T m =590 K. At sufficiently high I CP photo-induced attempts are dominant and generate local T ~800 K, independent of I CP . The fitted scaling (barrier attack) times τ t =τ th , and τ t = τ ph ( I CP ) are shown as diamonds. The decays are bimodal in the ‘crossover’ regime where the thermal and photo-induced trial times are comparable, with the solid cyan lines calculated from the relaxation model generalized for bimodal behaviour ( Supplementary Equation S17 ). Vertical orange lines denote F A =1 pa/mol. ( c ) Average inverse rate τ t for successful local molecular orientational barrier crossings and therefore for tests of the collective barriers to orientation, as a function of incident CP light intensity I CP . At low I CP , τ t has its thermal value ( τ t =τ th ~2 s), requiring ~10 11 room temperature molecular fluctuations to overcome a T th ~7,500 K local barrier, while at high I CP we find τ t ~ τ ph ( I CP ), which is nearly equal to (1 pa/mol)/ I ACP , where I ACP is the absorbed CP intensity ( Supplementary Note 1 , Supplementary Equation S2 ). This indicates that on average every absorbed photon generates a local barrier crossing test, evidence for a glass (fluidization) transition that obliterates the local barrier. This photo-induced bypass of the thermal trial process is responsible for the orientational photo-fluidization by CP illumination, directly manifested here as an orientational viscosity that decreases inversely with increasing intensity ( γ 1/ I CP ). Full size image This slow thermal relaxation is indicative of an activated, barrier-limited decay process, as typically described by an Arrhenius law, τ ( )= τ r exp( / k B T ), where 1/ τ r is the rate of barrier-crossing attempts on the molecular orientational fluctuation time scale, at most τ r ~20 ps [18] , is a barrier height and τ ( ) is the characteristic time of exponential relaxation, as sketched in Fig. 4a . However, the clearly nonexponential nature of the relaxations, shown explicitly in Fig. 2b , suggests that τ ( ) should be generalized to include a distribution of energy barriers, f ( ), a notion consistent with the heterogeneous nature of the monolayer, noted in (i) and (ii) above. The minimal decay for τ < τ t shows that f ( ) has a ‘barrier gap’, that is, little or no density of barriers below a minimum energy U t that can be estimated in the thermal case as U th / k B ≡ T th ~ln( τ th / τ r ) T ~ln(10 11 ) T ~25*300 K~7,500 K, a large value, likely due to the monolayer density and the tether constraints. It is therefore useful to write = U t + U , defining a density f ( U ) normalized in U , and the corresponding τ ( U )= τ r exp( U t + U )/ k B T = τ t exp( U / k B T ), with τ t = τ r exp( U t / k B T ). The inverse ‘trial’ time 1/ τ t (~0.5 Hz for thermal decay), obtained from the trial barrier U t , then serves as the rate for attempts to cross barriers distributed with f ( U ). Writing Q ( t )=∫ g ( t / τ ) H ( τ ) dτ , where the distribution of relaxation times τ ( U )= τ t exp( U / k B T ) is H ( τ ( U ))= f ( U )/|d τ ( U )/d U| , gives a relaxation of the form Q ( t )= G ( t / τ t ), showing that it is the barrier attack trial time τ t that becomes the scaling time for the relaxation ( Supplementary Note 5 ). For generality, we have assumed that the relaxation dynamics of the order parameter for each τ mode or event is stretched exponential, Q τ ( t )=exp-( t / τ ) α . However, the mode dynamic exponent α is found to significantly affect only the photo-writing dynamics. 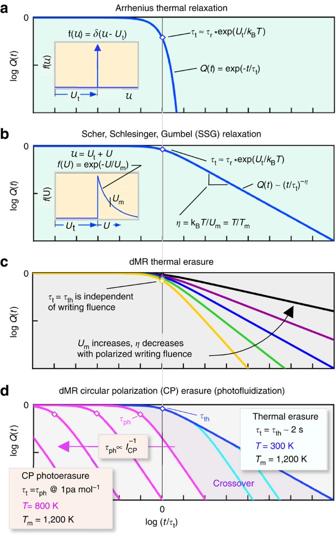Figure 4: Summary of relaxation processes relevant to the dMR SAM. (a) A delta function distribution of barrier heights,f(U)=δ(U—Ut), results in an Arrhenius thermally activated relaxation for which the decay function is exponential in timeQ(t)=exp(−t/τt),with scaling timeτtdetermined by the barrier gap,Ut, and a molecular fluctuation rateτr−1. (b) Decay for an orientational glass of local domains stabilized by a minimum local energy barrierUt, with collective interdomain interactions giving an additional energyU, distributed exponentially at largeU,f(U)=exp(−U/Um) as for the Scher/Shlesinger distribution43shown here. The result is a decay function with a ‘corner’ atτtdetermined byUt, and a power law asymptotic decayQ(t)=(t/τt)−ηdetermined by exponentη=kBT/Um. (c) In the thermally relaxing dMR SAM,Uthand thereforeτthare determined locally, in oriented glassy clusters of a few molecules originally created by single photon-induced isomerization events.Umincreases with enhanced collective interaction of such oriented clusters, so thatη=kB(300 K)/Umdecreases with increasing writing fluence. (d) In the CP photoerasure of the dMR SAM, the effective barrier attack temperature, also established in single photon-induced isomerization events, isTloc=800 K, melting the local collective glassy state and producing attacks on the barriers due to coupling to neighboring molecules with unit quantum efficiency. The faster power law decay that results,η=kB(800 K)/Um, is evidence that all barriers inf(U) are attacked atTeff=800 K, and thus that even the high energy barriers inf(U) are quite localized, necessarily within the 1 nm/10 psec space-time volume of a photoorientation event. Figure 4: Summary of relaxation processes relevant to the dMR SAM. ( a ) A delta function distribution of barrier heights, f ( U )= δ ( U — U t ), results in an Arrhenius thermally activated relaxation for which the decay function is exponential in time Q ( t )=exp(− t / τ t ),with scaling time τ t determined by the barrier gap, U t , and a molecular fluctuation rate τ r −1 . ( b ) Decay for an orientational glass of local domains stabilized by a minimum local energy barrier U t , with collective interdomain interactions giving an additional energy U , distributed exponentially at large U , f ( U )=exp(− U / U m ) as for the Scher/Shlesinger distribution [43] shown here. The result is a decay function with a ‘corner’ at τ t determined by U t , and a power law asymptotic decay Q ( t )=( t / τ t ) − η determined by exponent η = k B T / U m . ( c ) In the thermally relaxing dMR SAM, U th and therefore τ th are determined locally, in oriented glassy clusters of a few molecules originally created by single photon-induced isomerization events. U m increases with enhanced collective interaction of such oriented clusters, so that η = k B (300 K)/ U m decreases with increasing writing fluence. ( d ) In the CP photoerasure of the dMR SAM, the effective barrier attack temperature, also established in single photon-induced isomerization events, is T loc =800 K, melting the local collective glassy state and producing attacks on the barriers due to coupling to neighboring molecules with unit quantum efficiency. The faster power law decay that results, η = k B (800 K)/ U m , is evidence that all barriers in f ( U ) are attacked at T eff =800 K, and thus that even the high energy barriers in f ( U ) are quite localized, necessarily within the 1 nm/10 psec space-time volume of a photoorientation event. Full size image Pursuing the idea of a barrier height distribution, we have found that f ( U ) predicted from models of extreme value statistics, describing the density of the energies of the deepest minima in rough energy landscapes [35] , [36] , [37] , [38] , [39] , [40] , [41] , in particular those of the Gumbel university class [35] , provide an excellent description of our relaxations. Specifically, as first noted by Pfister and Scher, [42] and by Shlesinger [43] , the observed power law kinetics at large t emerge in a natural way if the high-energy tail of f ( U ) is exponential in the limit of large U , as also predicted from the extreme value statistics and Gumbel models [44] , [35] , [39] . The exponential tail distribution and its relaxation dynamics are outlined in Fig. 4b . The normalized Gumbel distribution ( Supplementary Note 5 ) where β is a parameter and Γ (1/ β ) is the gamma function, cuts off as a double exponential for U <0 to create a barrier gap, and is exponential at large U , f G ( U )~exp-( U/U m ), with decay constant U m the mean barrier height of the exponential tail. For β = α / η , f G ( U ) gives an effective distribution of relaxation times H G ( τ )=[ α /Γ( η / α ) τ t ] [exp-( τ t / τ ) α ] [ τ / τ t ] −( η +1) , which can then be integrated as written above to give the order parameter relaxation: Thus, the Gumbel H G ( τ ) yields a relaxation function which is simple but provides high-quality fits of our Δ n ( t ) relaxation data (magenta curves in Figs 2b and 3b ), where we take Q G ( t )=Δ n ( t )/Δ n (0). Q G ( t ) is scaled by τ t and at long time, where Q G ( t )<1, we have Δ n ( t ) Q G ( t ) ( t / τ t ) − η =( t / τ t ) − k T B / U m =( t / τ t ) − T/Tm , a power law time decay depending only on: (i) the parameter η , which is the decay exponent η = T / T m , governed by the ratio of the thermal activation energy k B T to U m = k B T m , the characteristic scaling energy of the exponential tail of the written barrier height distribution; and (ii) the barrier-crossing attempt rate 1/ τ t , which sets the time scale. The decay at long time is power law because in the course of a relaxation, once the barriers below some particular energy U ( t ) have been crossed, the average height of the remaining barriers is always U ( t )+ U m . In the Q G ( t ) fits, the time of the ‘corner’ on the log–log plots largely determines τ t , with fit values shown by diamonds in Figs 2 , 3 , 4 and by the data in Fig. 3c . The large- t slope largely determines η . The mode dynamic exponent is found to be α ~0.8, controlling primarily the initial writing, described by Δ n ( t ) 1— Q G ( t ) ( Fig. 2a and Supplementary Fig. S5 ). Our principal results emerge from the decay fits, as follows. SAM glassy relaxation: two distinct barrier-crossing processes We identify a local process that determines τ t and a collective process that increases η with increased writing fluence. We begin by discussing τ t , noting that the photo-writing and erasure proceeds by a series of discrete, random photon absorption events that, at the intensities used here (<1 kW cm −2 ), are widely separated in spacetime, a result of their short duration (~10 ps) and small spatial dimension (~1 nm Supplementary Note 5 ), as detailed in the discussion of isomerization events below. This can be seen from Fig. 3c , where the fraction of time an illuminated molecule spends in photo-events is plotted versus intensity, in this case for CP erasure. Thus, in the writing of an initially random state at low fluence, F A <1 pa/mol, the birefringence, which grows nearly linearly with time or F A ( Fig. 2a ), is the average measure of the local orientation of isolated groups of a few molecules, each orientation event induced by a single photon. The Q G ( t ) thermal decay fits in Fig. 2b , where τ t = τ th is found to be independent of writing fluence down to F A <1 pa/mol ( Fig. 2c ), combined with the data of the inset of Fig. 2a , which shows that the induced Δ n ( t ) depends only on fluence even for the slowest (low intensity) writing, indicate that the thermal lifetime of the isolated oriented few-molecule clusters in an otherwise random monolayer is τ th ~2 s in the F A <1 pa/mol regime. This clearly shows that the constraints determining τ th and thus U th are local. An estimate of a local orientational viscosity γ can be obtained by assuming orientational diffusion governed by the constant D = k B T /8 πγa 3 . Taking 1/D~τ th ~2 s and radius a ~0.5 nm yields γ ~10 8 poise, quantifying the glassy nature of dMR orientation. Turning to η , the Q G ( t ) fits of Fig. 2b show that for F A >1 pa/mol, where local areas experience multiple absorption events during writing, the decay exponent η increases with increasing F A . As the thermal erasure occurs at T ≈300 K, the behaviour of η = T / T m for the thermal decays shows that T m ( F A ) increases from 500 K to 1,200 K as F A increases from 0.5–250 pa/mol, evidence for an extension of the exponential tail of f ( U ) to higher energies, and thus a deepening of the barriers determining f ( U ). Fig. 2d shows that, at large F A , both T m ( F A ) and the written birefringence Δ n ( F A ) from Fig. 2a increase as log( F A ), indicating that incrementally enhanced written order produces incrementally deeper barriers. The enhancement of the very-deep barriers responsible for the power law tails at long times suggests a collective process originating in the mutual stabilization of local-oriented domains of a few molecules, which is enhanced as each locality experiences multiple orienting events in a temporally extended writing process. A molecule must overcome its local orientational barrier U th , which does not change significantly with F A , to make a test of the barriers given by f ( U ), which become deeper with increasing F A . Photoerasure cross-over to an intensity-independent elevated local T Once T m ( F A ) is known, Fig. 2b enables the comparison of the thermal and the CP decays for writing with F A =0.5, 12 and 60 pa/mol, and thereby a determination from η = T CP ( F A )/ T m ( F A ) of the effective temperature T CP for the circular polarized erasure, in this case at the erasing intensity I CP =1,000 mW cm −2 . The larger slopes for the CP case show that the effective temperature for attack of the f ( U ) barriers during CP erasure is larger than T =300 K. Calculating T CP from T CP ( F A )= ηT m ( F A ) gives similar effective erase temperatures, T CP =760 K, 710 K and 770 K for the three values of written F A common to the thermal and CP-erased relaxations, respectively. This constancy is evidence for the key result that the T m values and thus the barrier height distributions are the same for thermal and CP erasure. Taking T CP =750 K, we can then determine the barrier T m ( F A ) for the various F A values, up to T m ( F A =675 pa/mol)=1,670 K, which is not accessible thermally because the thermal decay becomes exceedingly slow for such large F A . Figure 3a and b shows series of relaxation curves of the dMR SAM orientationally written with fixed polarized writing fluence F A =1.25 pa/mol and erased with either thermally or with increasing intensity I CP of CP light. For thermal eraseure ( I CP =0, T =300 K), we measure η = T / T m =0.51, corresponding to a mean orientational barrier height T m =590 K induced by the F A =1.25 pa/mol writing. Fitting these data to Equation 2 yields trial times, τ t , shown for each curve in Figs 2b and 3a by the diamonds. Also shown is the time for which the absorbed fluence during erasure is one photon per molecule ( F A =1 pa/mol). For thermal erasure, τ th ≡ τ t ( I CP =0) is of order several seconds. τ t ( I CP ), shown in Fig. 3c , begins decreasing with increasing I CP in the cross-over regime where the photo-assisted trial rate becomes comparable to the thermal: τ t ( I CP ) ~ τ th . For I CP >~100 mW cm −2 , where τ t ( I CP ) << τ th , we label the photon-controlled asymptotic variation of τ t ( I CP ) as τ ph ( I CP ) in Figs 3a–c and 4d . In the τ t ( I CP ) ~ τ th cross-over regime ( I CP ~10 mW cm −2 ), the decays fit to a bimodal model (solid cyan curves of Fig. 3b ), with the thermal slope at short time and the photo-event slope at long time ( Supplementary Note 6 ). At high I CP , where τ t ( I CP ) < τ th , η saturates at an I CP -independent asymptotic value, η CP =1.50. This corresponds to an effective temperature T CP = η CP T m =890 K, which, according to our energy landscape model, is the temperature of the local structure as it makes trial attempts to overcome its orientational barriers. This is somewhat larger than T CP =740 K for the SAM of Fig. 2a , typical of the SAM-to-SAM variation of T CP , which in our data averages to T CP =800±100 K. The fact that temperature T CP becomes independent of I CP once it is large enough that the trials are predominantly photon generated shows that T CP is not related to the average energy flux. Rather T CP can be understood as an effective local temperature, a feature of local transient processes that are completely isolated spacetime events even at the highest intensities employed here. Figure 3c shows the variation of τ t with I CP , and we see that in the high I CP regime τ ph ( I CP ) varies as 1/ I CP (black dashed line) and is very close to τ t =(1pa/mol)/ I ACP (solid orange line), the time required for F A to grow to F A =1 pa/mol ( Supplementary Equation S2 ). This near equality indicates that the CP erase process has quantum efficiency, QELF ~1: one barrier escape trial per molecule is generated for each absorbed photon. Returning to our model above of relaxation as a local orientational diffusion limited by viscosity γ and noting also that γ τ t , we see immediately that the much more rapid decays induced by CP light ( Figs 2b and 3a ) due to the reduction of τ ph ( I CP ) with increasing I CP , is a manifestation of orientational photofluidization. In Fig. 3c we therefore also plot this behaviour as a photo-induced reduction of relative viscosity γ ( I CP )/ γ (0), with viscosity reduction by a factor of ~10 −5 found already at the relatively modest laser intensity of 1 kW cm −2 . Figure 3c then shows directly that the key signature of this photofluidization is a cross-over with increasing I CP to a viscosity that is inversely proportional to light intensity. Because of the low density of events in spacetime (top axis), the illumination produces no detectable average heating, that is, the fluidization is ‘athermal’. Photoabsorption/isomerization events Absorption of a photon at 514 nm deposits an energy of hν =2.4 eV into a dMR azo core, enough to excite a single harmonic degree of freedomto =29,000 K. Some fraction of this energy appears in a form that locally tests the molecular orientational barrier distribution at the effective temperature of T CP ~800 K. Fast spectroscopy [45] , [46] , [47] , quantum/molecular dynamic simulation [18] , [48] and molecular dynamic simulation [17] provide a semi-quantitative picture of this process, indicating that it is principally mechanical, with the photon energy appearing as a coherent force acting transiently on the environment of the absorbing molecule [49] , [50] , as follows. Upon photon absorption and electronic excitation, the azo core returns to the ground electronic manifold in a transition state configuration from which coherent change of the intra-molecular configuration takes place along one of several possible paths,for example, trans to cis or trans to trans , all of which reduce the internal potential energy by ~2 eV (45 kcal per mole), representing almost all of the absorbed photon energy [18] , [48] . For example, the transformation of the core from trans to cis is effected by a 180° change of the CNNC dihedral angle. In vacuum this transformation is a smooth slide down the ground state potential energy surface as a quasi-exponential damped relaxation (characteristic time=0.4 ps) [18] . In this process the vibrational modes of the molecule are thermalized, with the energy ending up principally in the fully excited low-frequency vibrations and the molecule which reach an internal temperature of ~1,100 K [45] . However, in solution nearly all of the energy of such a coherent change of molecular shape is released as orientational and translational work done on neighbouring molecules [18] , [47] , [48] . In particular, the detailed simulations of Tiberio et al. [18] show that for azobenzene in solvent, changes in molecular shape are predominantly opposed by intermolecular viscous forces rather than by intramolecular dissipation, leading to a damped relaxation on a much longer time scale (~>10 ps) than in vacuum, a dynamic to be expected ( Supplementary Note 7 ) and confirmed by experiment [46] . In this circumstance the decay becomes too slow to excite molecular vibrations and the potential energy of the azo goes mostly into inducing coherent motion of the solvent, as well as rotation and translation of the azo core. The 2 eV energy released corresponds to ~30 harmonic degrees of freedom at 800 K with which to attack the molecule’s orientational barriers. The fact that the quantum efficiency for barrier trials, QE ~1, is larger than that for trans – cis isomerization (0.3< QE trans-cis <0.7) [9] is an indication that the absorbed photon energy is deposited into the neighbours of an excited molecule, regardless of whether it makes it to cis or returns to trans [18] . The MD simulations of Teboul et al. [17] , [51] also show localized transient enhancement of mean square molecular displacement and dynamical heterogeneity in clusters surrounding isomerizing molecules. However, these simulations are difficult to use directly because the net energy deposited is not reported. Photofluidization: a glass transition of the local barriers This analysis shows that in a dense medium, photon-induced molecular shape change of the azo core occurs on the 10 ps time scale, sufficiently slow that it produces a coherent force transient on neighbouring molecules (as opposed to molecular vibrations [49] , [50] ), depositing ~2 eV of mechanical energy, enough to produce an orientational event with an effective local temperature of T =800 K. If only rotations about short molecular axes were so excited (an unlikely occurrence), then an upper estimate of ~30 molecules could be directly involved. As, in general, there are translational, other rotational and low-lying vibrational modes that will also be excited, the actual number of participating molecules must be smaller, probably limited to groups of nearest neighbours (~7 molecules). As noted above, the initial writing leaves such a group with a barrier of U th ~ k B (7,500 K) for reorientation. With this barrier and a photo-induced attack temperature of T =800 K, the number of photon absorption events to generate a trial would be exp[7,500K/800K], that is, a QELF <10 −4 , orders of magnitude less than the observed QELF ~1. This comparison implies that there must be a glass fluidization transition in the local barrier-crossing process at temperatures between 300 and 800 K, yielding a much smaller effective barrier at an attack temperature of T =800 K than at T =300 K. The experiments do not produce direct information on the nature of this transition, but its existence is not surprising, as T =800 K exceeds the glass transition temperature ( T g ) of most organic media, and simulation evidence for induced dynamic heterogeneity in an azo-doped polymer system has been reported [51] . The T loc =800 K local, photo-driven trial temperature therefore melts the collective local structures, possibly few molecule H- or J- aggregates, that are constraining reorientation to enable a group of molecules to execute a ‘trial’ test at T loc =800 K of the barriers coming from the coupling to neighbouring oriented molecules. The small fraction of time that a molecule is taking part in an event, shown in Fig. 3c for the intensities used here, guarantees that photofluidization is produced by a stream of randomly-occurring, isolated, discrete photo-orientation events. In each of these events T loc =800 K competes with a reorientation barrier U , distributed from site-to-site with f ( U ). This competition is a process involving the collective behavior of a molecule and only its nearest neighbors since, as discussed in the previous section, only a few molecules can be heated transiently to this temperature. Such a stream of random photo-orientation events encountering an exponentional distribution of barrier heights produces the observed power law decays. In this circumstance, the local glass transition in which a group of a few molecules ‘melts’, reorients and ‘refreezes’ is clearly a mechanism for the kind of permanent macroscopic (shape) change found in azo-based sytems [17] , [14] . Writing at large F: coupled aging of order and mean barrier height The slow aging shown in Fig. 2d , with Δ n ( F A ) and T m ( F A ), increasing as ln F A with F A in the range 10< F A <10 4 pa/mol, indicates a barrier-limited writing process. The barriers encountered in writing are just those that are established and must be overcome in reverse during erasing, that is, the characteristic energy scale for writing is T m . Then, assuming a photo-generated trial frequency, ν w , for writing (for overcoming the barriers to achieve an oriented state), the energy scale written at time t is given simply by the ‘exhaustion’ condition, defining δU m ( t ) to be the energy boundary between the low barriers that on average have already been crossed at time t ( P ( t )>1) and the high ones yet to be crossed [52] : 1≈ P ( t )= tν w exp(− δU m ( t )/ k B T ). Solving for δT m ( t ) gives δT m ( t )≈ T ln( tν w ) or δT m ( t )≈ T ln( F A / F A w ), where F Aw is the fluence required for a writing trial. From Fig. 2d , at F A =10 3 pa/mol we have δT m / T ≈4.3, giving F / F w =74 and therefore F w =14 pa/mol as the trial rate for writing expressed as a fluence absorbed by an isotropic sample (the actual absorbance will be around half of this value because of the orientational ordering induced). In this asymptotic regime, each molecule must therefore be put through the trans – cis – trans cycle ~10 times to generate a trial whereby further polarized illumination can enhance coupling between local glassy domains to increase T m . While single writing photons efficiently create local glassy oriented domains, it takes many writing photons to link them together to establish both better order and a barrier distribution having a tail extending to higher energies. This coupling of order and barrier height can also be understood as an example of orientational work hardening ( Supplementary Note 8 ) [52] . The high temperature and the resulting high quantum efficiency of photo-induced local barrier attack resulting from azo isomerization enables an understanding of the ability of photo-isomerization to reduce the viscosity of structural glassy hosts with only a tiny fraction of the average temperature increase that would otherwise be required [4] , [14] , [5] . For example, CP illumination of a T =300 K azo side-chain polymer glass, 120 K below its T g , produces negligible mean temperature increase (~<1 K) but reduces the viscosity of the mixture by several orders of magnitude, a change that, if produced by average temperature rise, would require heating to T g ~400 K [4] , [6] . The requirement for this kind of viscosity reduction also emerges in the fitting of theoretical descriptions of azo-based photo-manipulation to data describing permanent shape change effects induced by light, the latter behaving as if the average temperature had actually increased [4] , [5] , [6] , [14] , [53] . Illumination produces a stream of randomly occurring photon absorption events, each of which induces a local glass transition, a fluidization event that melts the local barrier, enabling attack of the barriers from coupling to neighboring molecules with unit quantum efficiency and high temperature. The work presented here leads us to propose that photofluidization arises in 3D structural glasses for the same reason. In structural glasses, including the host polymers for azo dyes [4] , the process corresponding to the dMR SAM orientational decay is the α structural relaxation, characterized by a Kohlrausch– Williams–Watts (KWW) stretched exponential decay of order q ( t ) exp(− t / τ α ) β and a relaxation time scale τ α that diverges upon cooling towards the glass transition. A variety of models have been put forth to describe this kind of relaxation [54] , each with a process producing the KWW temporal form and each with a distinct interpretation of the physical origin of τ α . Our results on the dMR SAM show that discrete local energy deposition events, which produce efficient high-temperature barrier attacks effectively, operate in parallel with and can thus ‘short out’ the thermal process determining τ t . This experimental fact in and of itself shows that the proper interpretation of τ t must be as an inverse rate of attack of the coupling to neighboring molecules that gives the exponential tail of the distribution, and the analogous observation of photofluidization in structural glasses shows that the same should be true for τ α . This is the case in, for example, the model in which structural relaxation is mediated by the diffusion of mobile defects limited by barriers with an exponential distribution of barrier heights of mean height T m and attack trial time τ α [43] . In this model, the one most closely related to that used above to describe the dMR SAM, the temporal behaviour and the decay exponent, in this case β=T/T m, are determined by the distribution of barrier heights encountered once a barrier attack is achieved. For the dMR SAM the decay curves of CP light erasure and thermal erasure are quantitatively of the same form and have the same ( T m ) scaling behavior. This leads us to suggest that the overall reorientation process is the same in the two cases: a fluctuation corresponding to a local melting of a cluster of a molecule and a few of its neighbors that encounters a distribution of barriers against reorientation. This process occurs for every photon absorbed but only rarely at room. Photofluidization of bulk polymers indicates that the same may be the case for structural glasses, which could be tested by study of relaxation dynamics of azo-containing systems in the presence of unpolarized actinic light. Key tests of the ideas presented here would be made possible by finding a way of tuning the amount of deposited energy. Any azo system that absorbs incident light will deposit local energy bursts, but the effectiveness of this energy in producing local structural deconfinement, and the nature of the glassy behaviour itself, will depend on the details of molecular structure, interactions and tethering. Molecules from other azo-based cores that are similarly tethered into monolayers [11] , and in-situ structural manipulation of the monolayers, by mixing or photochemistry, for example, are also of great interest. High-sensitivity polarimeter A high extinction polarimeter as shown in Supplementary Fig. S1 has been employed to measure the tiny birefringence changes in the SAMs induced by exposure to polarized light [21] . The polarimeter uses a 0.7-mW helium–neon laser focused to a 40-μm diameter spot on the sample as the probe beam, achieving a static (DC) minimum transmission ratio T min = I ┴ / I || =2.4 × 10 −10 , where I ┴ , I || are the transmitted intensity between the crossed and parallel polarizer and analyser, respectively. Supplementary Figure S2 shows the extinction minimum as the analyser is very slightly uncrossed. For an anisotropic organic monolayer between air and a substrate of index n g , illuminated with visible light, the retardance is very small and the transmission T is well approximated by where a principal optic axis is along the mean in-plane molecular long axis orientation of the monolayer n , θ is the angle between n and the polarization of the probe light, d =0.5 nm is the film thickness, n g =1.5 is the index of refraction of the glass substrate, n m =( n || + n ┴ )/2 is the mean index of the SAM film, estimated to be n m ≈1.6, and λ =633 nm is the probe light wavelength (see Supplementary Methods ). When θ is set to=45° to get the maximum transmission, the birefringence Δ n can be obtained approximately as Δ n ( λ / πd) ( T ) 1/2 , where we have taken 4 n m /( n g +1) 2 1. dMR synthesis The methyl red derivative shown in Fig. 1 , 2-[(1E)-2-[4-(dimethylamino)phenyl]diazenyl]- N -[3-(triethoxysilyl)propyl]-benzamide [19] , is synthesized through a 1,3-dicyclohexylcarbodiimide (4.77 g) coupling between methyl red (5.75 g) and 3-aminopropyltriethoxysilane (4.73 g) in solvent of dichloromethane (60 ml). The dichloromethane is distilled from CaH 2 . The reaction is carried out overnight, stirring under argon. The resulting solution is filtered and concentrated to form dark red oil. Dark red crystals are obtained by purifying this oil using silica gel column chromatography (50% ethyl acetate, 50% hexane). Glass cleaning The glass substrates used here were cleaned using ‘piranha’ solution composed of 1:1 concentrated H 2 SO 4 : 30% H 2 O 2 . Substrates are soaked in the piranha solution for 1 h, then sonicated and rinsed in distilled deionized water several times, and blown dry with pure nitrogen gas. The cleaned substrates are hydrophilic and were checked to be cleaned well by requiring complete wetting of deionized water. The hydrolysed surfaces are used to form covalent bonds with the triethoxysilane group in dMRs. Monolayer formation The preparation of the SAMs is carried out as follows: 272 mg of dMR is dissolved in 70 ml of toluene with 0.25 ml n -butylamine as a catalyst. The resulting solution is heated to about 45 °C while being sonicated to form a homogeneous solution. A clean, dry glass substrate is put into the solution, which is further sonicated to prevent molecules from physically attaching to the glass. After 90 min, the substrate is taken out of solution and rinsed with toluene until the toluene does not absorb any more colour from the glass substrate. Finally the substrate is blown dry with pure nitrogen and cured at 115 °C in vacuum for 1 h. Azo-SAM Cells Azo-SAMs photo-oxidize if they are exposed to air and light concurrently. Therefore, all experiments reported here were carried out using sealed cells made from pairs of SAM-coated substrates ( Supplementary Fig. S3 ), with the azo-SAMs on the inner glass surfaces bathed in an inert argon atmosphere. Epoxy was used to seal the periphery, and the azo-SAM monolayers on the outer glass surfaces were then removed using piranha solution. Such cells were employed to measure the reorientation dynamics of bare monolayers using the precision polarimeter described above. Background birefringence The polarimeter reveals that stress-induced birefringent phase shifts at a randomly chosen place on the glass microscope slide substrates can be large compared with that of the monolayer. To avoid this problem it is necessary to first scan the glass birefringence with the monolayer thermally randomized to find a position on the glass with minimum transmitted intensity (a line where the birefringence of the glass is changing sign), which is typically mostly from the polarimeter leakage. This leakage, which appears as the asymptotic background at long time in the relaxations Fig. 3 , is stable in intensity in a given experiment over periods of hours. The thermal relaxation of the monolayer to an isotropic state enables this background to be counted over extended periods and subtracted out. How to cite this article: Fang, G.J. et al. Athermal photofluidization of glasses. Nat. Commun. 4:1521 doi: 10.1038/ncomms2483 (2013).